Gene pleiotropy constrains gene expression changes in fish adapted to different thermal conditions Understanding the factors that shape the evolution of gene expression is a central goal in biology, but the molecular mechanisms behind this remain controversial. A related major goal is ascertaining how such factors may affect the adaptive potential of a species or population. Here we demonstrate that temperature-driven gene expression changes in fish adapted to differing thermal environments are constrained by the level of gene pleiotropy estimated by either the number of protein interactions or gene biological processes. Genes with low pleiotropy levels were the main drivers of both plastic and evolutionary global expression profile changes, while highly pleiotropic genes had limited expression response to temperature treatment. Our study provides critical insights into the molecular mechanisms by which natural populations can adapt to changing environments. In addition to having important implications for climate change adaptation, these results suggest that gene pleiotropy should be considered more carefully when interpreting expression profiling data. The significance of gene expression pattern modification as a component of the adaptation process has received considerable attention recently [1] , [2] , [3] , [4] . Gene expression has been connected to many facets of evolution, either via adaptive changes or by plastic responses [5] , including population divergence in natural systems [6] , [7] , [8] and human populations [1] , sexual dimorphism [9] , [10] , sex chromosome evolution [10] , [11] , speciation [12] , [13] , as well as community and eco-evolutionary dynamics [14] . Despite this, several key questions regarding gene expression adaptation remain open [3] . First, whether or not gene expression changes tend to be neutral, or affected by natural selection, remains a point of contention [3] , [7] , [13] , [15] . Recent efforts have focused on refining models of gene expression evolution to better assess gene expression adaptation [1] , [3] , [16] , including application of a Q ST − F ST framework [7] , [17] , but several key questions regarding gene expression adaptation remain unanswered [3] . For example, gene expression evolution is typically driven by regulatory mutations as revealed by studies of genome-wide adaptive gene expression variation [1] , [2] , [3] , [4] , [18] , [19] ; however, a mechanistic framework for understanding how gene expression evolution leads to modified biological function and phenotypic adaptation is still underdeveloped in evolutionary and molecular biology. One approach to address this problem is to view gene expression evolution in the context of the interactome, the complex network of all molecular interactions [20] . Biological function is rarely the property of single gene products, but rather is carried out by proteins that cooperate with each other often at stoichiometric ratios. As a consequence, interacting proteins have expression profiles that tend to co-evolve [21] . What factors, if any, can influence gene expression evolution in the protein interaction network is, however, unknown. The importance of pleiotropy, that is, when one locus affects multiple phenotypic characters, has been an active topic of discussion in evolutionary biology for many years and remains controversial [22] , [23] . At the molecular level, pleiotropy and predictions of its consequences are generally built within the framework of Fisher’s geometric model, also summarized as the ‘cost of complexity’, which predicts that complexity associated with pleiotropy will constrain adaptive evolution [24] , [25] , [26] . Gene pleiotropy has been found to positively correlate with the number of biological processes or protein–protein interactions (PPI) in which a gene is involved, but not with the number of molecular functions [27] . Pleiotropy at the molecular level is thus the result of single molecular functions involved in multiple biological processes through interactions with other gene products. Historically, this has been called type II pleiotropy with the alternative hypothesis being that molecular pleiotropy is conferred by multiple molecular functions of a gene product (type I pleiotropy) [26] , [27] . Under this view, several studies have highlighted the importance of gene pleiotropy as a constraining factor in the rate of molecular evolution and in gene expression variation. For example, proteins with more interactions were found to have slower amino acid substitution rates in Saccharomyces [28] , [29] , [30] , Caenorhabditis [30] and Drosophila [30] . Further, they have been found to show lower interspecific gene expression divergence in Saccharomyces and Drosophila , as well as lower population-level gene expression variation [31] . Gene pleiotropy, as estimated by number of PPI, may thus have a role in gene expression evolution but more research is required to clarify this relationship. Key questions in particular that have yet to be addressed empirically are how gene pleiotropy affects gene expression evolution in varying environmental conditions and whether pleiotropy constrains adaptation at the gene expression level. We study a metapopulation of European grayling ( Thymallus thymallus ), a spring-spawning, freshwater salmonid fish with high homing propensity that has undergone contemporary evolution of early life-history traits in response to temperature [32] , [33] . Fish colonized Lesjaskogsvatnet (62°14′N 8°25′E), a lake in southern Norway, following an upstream watercourse manipulation in the late 1880s (≈25 generations) and subsequently established spawning sub-populations in tributaries with contrasting thermal characteristics, namely warmer versus colder relative to each other [33] , [34] ( Fig. 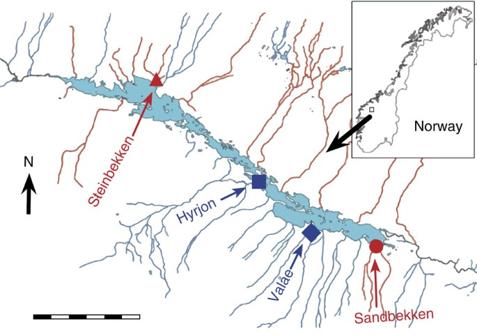Figure 1: Map of Lesjaskogsvatnet in Norway and the sampling locations of the sub-populations. Blue and red colour indicates cold and warm thermal origin, respectively. Scale bar, 3 km. 1 and Supplementary Table 1 ). 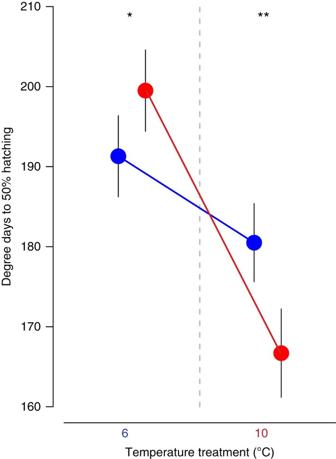Figure 2: Development rates of grayling juveniles in the common garden experiment. Degree-days (temperature in °C × number of days elapsed since egg fertilization) to 50% of the eggs to hatch were higher for the grayling in the cold temperature treatment. However, within a given temperature treatment, ‘local’ grayling hatched significantly earlier than ‘non-local’ grayling.P-values for differences in hatching time between populations within a temperature treatment were calculated using hatching data pooled per thermal origin of sub-populations (Binomial logistic regression: *P<0.05; **P<0.01. 6 °C:ncold=380,nwarm=549; 10 °C:ncold=234,nwarm=215). Blue and red colour indicates cold and warm thermal origin, respectively. Error bars represent s.e. Earlier research has provided convincing evidence that rapid adaptation of early life-history traits to differing thermal conditions has occurred in just 25 generations [32] , [33] , despite low effective population sizes, low levels of genetic divergence and variability at assumedly neutral molecular markers [33] , [35] , [36] ( Supplementary Table 2 ). As such, regulatory evolution leading to differences in gene expression is a likely to be a molecular mechanism driving the observed adaptations [4] . Figure 1: Map of Lesjaskogsvatnet in Norway and the sampling locations of the sub-populations. Blue and red colour indicates cold and warm thermal origin, respectively. Scale bar, 3 km. Full size image Here we show that gene pleiotropy has a constraining effect on protein expression change in European grayling sub-populations adapted to different thermal environments. We first confirm that juvenile grayling development rates conform to those expected under the local adaptation hypothesis using a common garden experiment with temperatures resembling the alternative natal environments. Next, using samples collected from the same experiment, we employ high-resolution mass spectrometry and measure gene expression directly at the protein level from embryos of similar developmental stage from both temperature treatments. We describe the general effect of gene pleiotropy on protein expression profiles following adaptation rather than providing a list of specific candidate genes responsible for the adaptations. We find that the global proteomic thermal profiles include both plastic and evolutionary components, and that protein expression responses negatively correlate to the level of gene pleiotropy. Development supports the local thermal adaptation hypothesis Grayling development rates in the common garden experiment were faster in the temperature most resembling the natal environment. Time to hatch was consistently longer in the cold temperature treatment. However, within a given temperature treatment, ‘local’ grayling, that is, grayling whose thermal origin was most similar to the temperature treatment, hatched significantly earlier than ‘non-local’ grayling ( Fig. 2 ). In the 6 °C treatment, 50% of cold thermal origin embryos were estimated to hatch on average 8.2 degree-days before 50% of warm thermal origin embryos had hatched (Binomial logistic regression: P =0.025, cold: n =380, degree-day 50% =191.3, s.e.=2.53; warm: n =549, degree-day 50% =199.5, s.e.=2.54). In the 10 °C treatment, 50% of warm origin embryos hatched on average 13.8 degree-days earlier than cold origin grayling (Binomial logistic regression: P =0.0012, cold: n =234, degree-day 50% =180.5, s.e.=2.44; warm: n =215, degree-day 50% =166.7, s.e.=2.76) ( Fig. 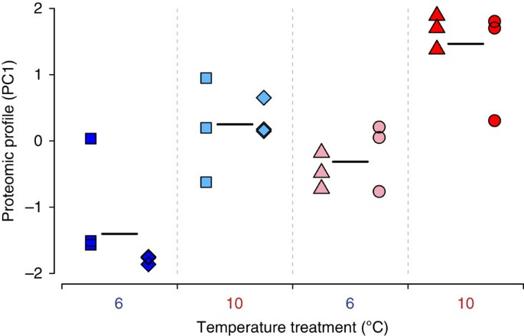Figure 3: Global proteomic profiles of grayling juveniles raised in the common garden experiment. An overview of individual grayling protein expression profiles on the first principal component (PC1: 36.7% of the variance in expression level of the quantified proteins). The GLMM revealed a highly significant effect of temperature treatment on protein expression profiles (plastic component; GLMM, type II Wald’s F tests with Kenward–Roger df:P=8.4E−07, F=53.68, df=1, df.res=18,n=24), a significant effect of thermal origin on protein expression profiles (evolutionary component;P=0.039, F=24.22, df=1, df.res=2,n=24) and no interaction between them (P=0.790, F=0.07, df=1, df.res=18,n=24). Symbols indicate different sub-populations and colours reflect thermal origin and temperature treatment (blue=cold thermal origin −6 °C, light blue=cold thermal origin −10 °C, pink=warm thermal origin −6 °C, red=warm thermal origin −10 °C). Lighter colours indicate ‘non-local’ origin-treatment combinations. Black-coloured horizontal lines represent the average over all six biological replicates of the same thermal origin within a temperature treatment. These results are based on the 244 proteins with no missing values. 2 and Supplementary Table 3 ). As rapid development has been shown to provide fitness benefits in salmonid fishes [37] , these results represent an archetypal case supporting the local adaptation hypothesis [38] . Figure 2: Development rates of grayling juveniles in the common garden experiment. Degree-days (temperature in °C × number of days elapsed since egg fertilization) to 50% of the eggs to hatch were higher for the grayling in the cold temperature treatment. However, within a given temperature treatment, ‘local’ grayling hatched significantly earlier than ‘non-local’ grayling. P -values for differences in hatching time between populations within a temperature treatment were calculated using hatching data pooled per thermal origin of sub-populations (Binomial logistic regression: * P <0.05; ** P <0.01. 6 °C: n cold =380, n warm =549; 10 °C: n cold =234, n warm =215). Blue and red colour indicates cold and warm thermal origin, respectively. Error bars represent s.e. Full size image Expression profiles have plastic and evolutionary components We tested the effect of temperature treatment, that is, 6 °C versus 10 °C, on the global protein expression profiles, and of thermal origin, that is, cold versus warm sub-populations. For this, we summarized the expression values of the 408 quantified proteins remaining after filtering (790 proteins were identified in total) along the first component (PC1) of a principal component analysis (PCA) and analysed the PC1 values with a general linear mixed model (GLMM). We found a highly significant effect of temperature treatment on protein expression profiles and a significant effect of thermal origin but no interaction between them ( Fig. 3 and Supplementary Fig. 1 ). In other words, we observed a strong plastic component, that is, expression change between different temperature treatments in samples of the same thermal origin, as well as an evolutionary component, that is, expression difference between samples of differing thermal origin in the same temperature treatment, with each component having an independent effect on the grayling protein expression profiles. Figure 3: Global proteomic profiles of grayling juveniles raised in the common garden experiment. An overview of individual grayling protein expression profiles on the first principal component (PC1: 36.7% of the variance in expression level of the quantified proteins). The GLMM revealed a highly significant effect of temperature treatment on protein expression profiles (plastic component; GLMM, type II Wald’s F tests with Kenward–Roger df: P =8.4E−07, F=53.68, df=1, df.res=18, n =24), a significant effect of thermal origin on protein expression profiles (evolutionary component; P =0.039, F=24.22, df=1, df.res=2, n =24) and no interaction between them ( P =0.790, F=0.07, df=1, df.res=18, n =24). Symbols indicate different sub-populations and colours reflect thermal origin and temperature treatment (blue=cold thermal origin −6 °C, light blue=cold thermal origin −10 °C, pink=warm thermal origin −6 °C, red=warm thermal origin −10 °C). Lighter colours indicate ‘non-local’ origin-treatment combinations. Black-coloured horizontal lines represent the average over all six biological replicates of the same thermal origin within a temperature treatment. These results are based on the 244 proteins with no missing values. Full size image The expression profiles were generally very consistent between the replicate sub-populations of different thermal origin in both temperature treatments. For instance, hierarchical clustering of normalized protein expression levels grouped cold and warm sub-populations separately when reared in the natal-resembling temperature ( Supplementary Fig. 2 ). The congruity of expression profile between the replicate populations, combined with the very recent divergence time (25 generations) of the sub-populations indicate that adaptation to the natal environment (either cold or warm streams) may have played a significant role in the evolution of their expression profiles. To investigate this further, we compared the level of protein expression divergence between cold and warm thermal origin sub-populations to the level of genetic divergence at assumedly neutral microsatellite markers using a Q ST − F ST framework [17] with a view to determining whether the null hypothesis of neutral evolution could be rejected. The mean Q ST between sub-populations was 0.086 and 0.076 for the cold and warm temperature treatments, respectively, which is four to five times higher than the mean F ST that was 0.017. Further, 139 (cold temperature treatment: 34.1%) and 124 (warm temperature treatment: 30.4%) of the 408 proteins analysed had Q ST values larger than the upper bound of the F ST 95% confidence interval, which is highly significantly more than expected by chance ( χ 2 -test: cold temperature treatment: P <1.00E−16, χ 2 =145.0, df=1, n =408; warm temperature treatment: P <1.00E−16, χ 2 =122.2, df=1, n =408). These findings thus suggest that the observed differences in expression levels between cold and warm origin sub-populations, that is, the evolutionary component of protein expression profiles, also include a strong adaptive component. Gene pleiotropy constrains protein expression responses We then tested the effect of gene pleiotropy on the plastic and evolutionary components of the protein expression profiles using a GLMM that also incorporated gene pleiotropy as an independent variable. For gene pleiotropy, we used the two alternative estimators, Gene Ontology (GO) and PPI, assigned to the human orthologues of the 408 proteins quantified in our experiment. The three GO categories, biological process (GO-BP), molecular function (GO-MF) and cellular component (GO-CC), were tested independently. We found a highly significant effect of the interaction between gene pleiotropy and thermal origin, and the interaction between gene pleiotropy and temperature treatment when gene pleiotropy was estimated as either PPI or GO-BP but not with GO-MF or GO-CC ( Fig. 4 and Supplementary Figs 3 and 4 ). 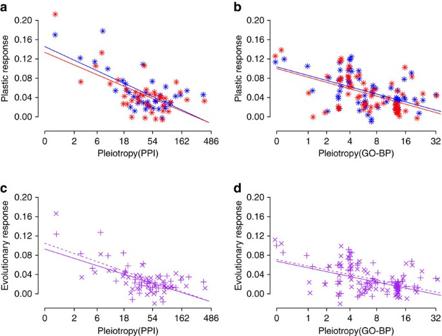Figure 4: Constraining effect of gene pleiotropy on plastic and evolutionary protein expression responses. (a,b) Plastic response of protein expression is represented as the difference in mean protein expression level between 6 °C and 10 °C temperature treatments in grayling of cold (blue colour) and warm (red colour) thermal origin. (a) Pleiotropy estimated by PPI: GLMM, type II Wald’s F tests with Kenward–Roger df:P=1.04E−25,n=960, bootstrap support=100%. (b) Pleiotropy estimated by GO-BP:P=4.99E−05,n=960, bootstrap support=81%. (c,d) Evolutionary response in protein expression represented as the difference in mean protein expression level between grayling of cold and warm thermal origins in the 6 °C (× symbol, continuous line) and 10 °C (+ symbol, dashed line) temperature treatment. (c) Pleiotropy estimated by PPI:P=7.05E−10,n=960, bootstrap support=93%. (d) Pleiotropy estimated by GO-BP:P=1.04E−04,n=960, bootstrap support=76%.P-values for the plastic response represent the interaction between gene pleiotropy and temperature treatment, and for evolutionary response the interaction between gene pleiotropy and thermal origin. Mild jittering of the points along thexaxis was applied to improve plot clarity. Lines are linear regression fits used for visualization. These results derived from GLMM analysis on mean standardized protein expression levels of grouped proteins (bin=10 proteins). Figure 4: Constraining effect of gene pleiotropy on plastic and evolutionary protein expression responses. ( a , b ) Plastic response of protein expression is represented as the difference in mean protein expression level between 6 °C and 10 °C temperature treatments in grayling of cold (blue colour) and warm (red colour) thermal origin. ( a ) Pleiotropy estimated by PPI: GLMM, type II Wald’s F tests with Kenward–Roger df: P =1.04E−25, n =960, bootstrap support=100%. ( b ) Pleiotropy estimated by GO-BP: P =4.99E−05, n =960, bootstrap support=81%. ( c , d ) Evolutionary response in protein expression represented as the difference in mean protein expression level between grayling of cold and warm thermal origins in the 6 °C (× symbol, continuous line) and 10 °C (+ symbol, dashed line) temperature treatment. ( c ) Pleiotropy estimated by PPI: P =7.05E−10, n =960, bootstrap support=93%. ( d ) Pleiotropy estimated by GO-BP: P =1.04E−04, n =960, bootstrap support=76%. P -values for the plastic response represent the interaction between gene pleiotropy and temperature treatment, and for evolutionary response the interaction between gene pleiotropy and thermal origin. Mild jittering of the points along the x axis was applied to improve plot clarity. Lines are linear regression fits used for visualization. These results derived from GLMM analysis on mean standardized protein expression levels of grouped proteins (bin=10 proteins). Full size image Genes with low pleiotropy drive expression profile changes Based on the above result, we sought to confirm the expected restrictive effect of gene pleiotropy on the plastic and evolutionary responses to temperature treatment observed in Fig. 3 . For this, we separated the proteins into two groups, high and low pleiotropy, using the median values of PPI and GO-BP, and repeated the GLMM analysis of the PC1 values for each case. We found that genes with low pleiotropy were the main drivers of protein expression profile change due to thermal origin and temperature treatment ( Fig. 5 and Supplementary Fig. 5 ). 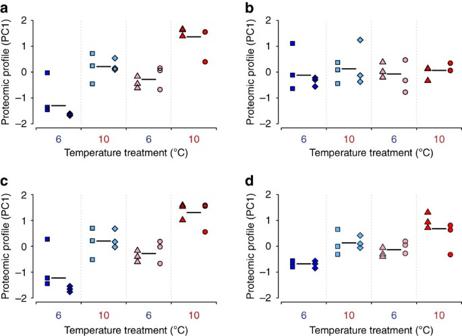Figure 5: Global proteomic profiles of genes with differing pleiotropy levels in grayling from the common garden experiment. Greater differences were observed for genes with lower pleiotropy levels than for genes with higher pleiotropy levels. (a) Low PPI. GLMM, type II Wald’s F tests with Kenward–Roger df:PPL=2.25E−07,n=24;PEV=0.03,n=24. (b) High PPI.PPL=0.37,n=24;PEV=0.80,n=24. (c) Low GO-BP.PPL=1.26E−06,n=24;PEV=0.04,n=24. (d) High GO-BP.PPL=2.04E−05,n=24;PEV=0.06,n=24. Significance was calculated using the PC1 coordinates in each case in a GLMM:PPLis the significance of the plastic component andPEVis the significance of the evolutionary component. PC1 described (a) 46.2%, (b) 22.2%, (c) 42.3% and (d) 29.2% of the variance. Symbols indicate different sub-populations and colours reflect thermal origin and temperature treatment (blue=cold thermal origin −6 °C, light blue=cold thermal origin −10 °C, pink=warm thermal origin −6 °C, red=warm thermal origin −10 °C). Lighter colours indicate ‘non-local’ origin-treatment combinations. Black-coloured horizontal lines represent the average over all six biological replicates of the same thermal origin within a temperature treatment. These results are based on the 244 proteins with no missing values. Figure 5: Global proteomic profiles of genes with differing pleiotropy levels in grayling from the common garden experiment. Greater differences were observed for genes with lower pleiotropy levels than for genes with higher pleiotropy levels. ( a ) Low PPI. GLMM, type II Wald’s F tests with Kenward–Roger df: P PL =2.25E−07, n =24; P EV =0.03, n =24. ( b ) High PPI. P PL =0.37, n =24; P EV =0.80, n =24. ( c ) Low GO-BP. P PL =1.26E−06, n =24; P EV =0.04, n =24. ( d ) High GO-BP. P PL =2.04E−05, n =24; P EV =0.06, n =24. Significance was calculated using the PC1 coordinates in each case in a GLMM: P PL is the significance of the plastic component and P EV is the significance of the evolutionary component. PC1 described ( a ) 46.2%, ( b ) 22.2%, ( c ) 42.3% and ( d ) 29.2% of the variance. Symbols indicate different sub-populations and colours reflect thermal origin and temperature treatment (blue=cold thermal origin −6 °C, light blue=cold thermal origin −10 °C, pink=warm thermal origin −6 °C, red=warm thermal origin −10 °C). Lighter colours indicate ‘non-local’ origin-treatment combinations. Black-coloured horizontal lines represent the average over all six biological replicates of the same thermal origin within a temperature treatment. These results are based on the 244 proteins with no missing values. Full size image No influence of potential biases in GO and PPI estimation We investigated whether our findings could be driven by biases (a) in the number of GO annotations from proliferating semantically similar terms that do not represent distinct GO-BP, GO-CC and GO-MF [39] or (b) in the PPI data set from the presence of few well-studied proteins for which many interactions have been reported [40] , [41] . For this, we repeated the analyses after summarizing the GO annotations assigned to each protein by grouping terms of similar meaning using different similarity thresholds [42] , [43] and performed bootstrap analysis on all data sets. We found that our observations remained unchanged and highly significant after GO summarization and had very strong bootstrap support, thus suggesting that it is unlikely our results are biased by these factors ( Supplementary Data 1 and 2 ). We further employed a spectral counting approach to obtain rough estimates of protein expression levels ( Supplementary Methods ) and found that the effect of gene pleiotropy remains very significant after expression level is taken into account ( Supplementary Fig. 6 ). This result further suggests that our findings are not due to any confounding factor linked to the expression level of the studied proteins [44] . Similar results using predicted PPI proxies in zebrafish To further validate our findings on PPI in the case of teleost fish, we used the results produced by an in silico method that predicts conserved PPI or interologs, that is, orthologous pairs of interacting proteins in different species [45] , [46] . Using zebrafish ( Danio rerio ) PPI proxies predicted with high confidence (>0.9) in the Funcoup database [47] , we found that the constraining effect of gene pleiotropy on both the plastic and evolutionary responses in grayling remained strong and significant ( Fig. 6 , Supplementary Fig. 7 and Supplementary Data 2 ). 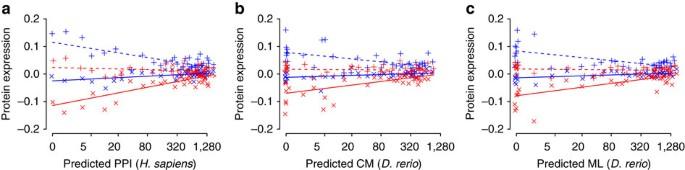Figure 6: The constraining effect of gene pleiotropy using predicted protein interactions. (a) Predicted PPI forH. sapiens. GLMM, type II Wald’s F tests with Kenward–Roger df:PPL=1.14E−30,n=960, bootstrap=100%;PEV=5.58E−14,n=960, bootstrap=99%. (b) Predicted CM forD. rerio.PPL=9.11E−10,n=960, bootstrap=98%;PEV=5.39E−05,n=960, bootstrap=85%. (c) Predicted ML forD. rerio. PPL=7.14E−18,n=960, bootstrap=99%;PEV=5.36E−09,n=960, bootstrap=95%.PPLis the significance of the plastic response andPEVis the significance of the evolutionary response in protein expression. PPI, protein–protein interactions; CM, coupling between proteins in the same complex; ML, coupling between proteins in the same metabolic pathway. Predicted PPI, CM and ML numbers were taken from the Funcoup 2.0 database47. CM and ML were used as predictors of PPI forD. rerio. Mild jittering of the points along thexaxis was applied to improve plot clarity. Lines are linear regression fits used for visualization. Continuous lines, × 6 °C temperature treatment; dashed lines, +10 °C temperature treatment; blue colour: cold thermal origin; red colour: warm thermal origin. Figure 6: The constraining effect of gene pleiotropy using predicted protein interactions. ( a ) Predicted PPI for H. sapiens . GLMM, type II Wald’s F tests with Kenward–Roger df: P PL =1.14E−30, n =960, bootstrap=100%; P EV =5.58E−14, n =960, bootstrap=99%. ( b ) Predicted CM for D. rerio . P PL =9.11E−10, n =960, bootstrap=98%; P EV =5.39E−05, n =960, bootstrap=85%. ( c ) Predicted ML for D. rerio . P PL =7.14E−18, n =960, bootstrap=99%; P EV =5.36E−09, n =960, bootstrap=95%. P PL is the significance of the plastic response and P EV is the significance of the evolutionary response in protein expression. PPI, protein–protein interactions; CM, coupling between proteins in the same complex; ML, coupling between proteins in the same metabolic pathway. Predicted PPI, CM and ML numbers were taken from the Funcoup 2.0 database [47] . CM and ML were used as predictors of PPI for D. rerio . Mild jittering of the points along the x axis was applied to improve plot clarity. Lines are linear regression fits used for visualization. Continuous lines, × 6 °C temperature treatment; dashed lines, +10 °C temperature treatment; blue colour: cold thermal origin; red colour: warm thermal origin. Full size image Upstream regulators link expression to phenotypic evolution To elucidate the biological causes and further explore the biological meaning of our observations, we searched for upstream regulators such as transcription factors that were predicted to have driven the observed gene expression changes [48] . We identified seven significantly activated or inhibited transcription factors in total, including hsf1 and hsf2 , and myc and mycn , out of 73 occurrences of transcription factors known to regulate the genes observed in our data ( Supplementary Table 4 ). We demonstrate empirically for the first time that gene pleiotropy constrains both plastic and evolutionary, presumably adaptive, components of gene expression change. We also reveal that genes with low levels of pleiotropy are of particular significance during the initial phases of evolution. Strong plastic and significant evolutionary components in the global protein expression profiles ( Fig. 3 ) give support at the molecular level for local adaptation of the grayling sub-populations, and furthermore, provide an ideal opportunity for elucidating the relative importance of plastic and adaptive responses during rapid fisherian evolution. The resulting significant effect of the interaction between either GO-BP or PPI and thermal origin and temperature treatment ( Fig. 4 and Supplementary Data 1 and 2 ) indicates an effect of gene pleiotropy on both plastic (interaction with temperature treatment) and evolutionary (interaction with thermal origin) protein expression responses. Differences in protein expression between experimental groups, that is, the extent of expression change, were also decreasing with increasing pleiotropic level for both plastic and evolutionary responses ( Fig. 4 ). These findings are consistent with Fisher’s prediction that pleiotropy restricts adaptation [24] , [25] , because trade-offs between changes in expression that favour one process but harm others are more likely to be in highly pleiotropic genes. These findings are also in concordance with the observation that genes with many genetic interactions confer robustness to environmental and stochastic change [49] . By comparison, genes with low pleiotropy had a stronger effect on both plastic and evolutionary responses ( Fig. 5 ), which indicates that genes with a low level of pleiotropy may play a particularly important role during the early phases of rapid evolution. At the interspecific level, Lemos et al . [31] observed a negative association between number of PPI and levels of gene expression variation in two Drosophila species. As such, the role of gene pleiotropy as described here may span a large range of evolutionary time scales. Our results on gene pleiotropy are in concordance with the current view that molecular-level pleiotropy is generally the result of a given molecular function being involved in multiple biological processes (type II pleiotropy) [26] , [27] . GO-MF had no significant effect on either plastic or evolutionary protein expression response ( Supplementary Figs 3 and 4 and Supplementary Data 1 and 2 ), which is contrary to what would be expected with type I pleiotropy. In the type II view of molecular-level pleiotropy, more biological processes have been further suggested to distribute to more cellular components [27] . In line with this finding, we observed a weakly significant association between GO-CC and both plastic and evolutionary gene expression responses ( Supplementary Figs 3 and 4 and Supplementary Data 1 and 2 ). By ensuring that the GO and PPI data sets yielded unbiased and meaningful results in European grayling, we also provide a general strategy for the use of this kind of information in non-model species. GO-BP annotations are well suited for cross-species use [50] , and correcting GO annotations for semantic similarity can help reduce biases in gene pleiotropy estimation coming from genes annotated with multiple terms for the same biological process [39] . This kind of annotation bias has earlier been a criticism of studies linking PPI and rate of evolution [40] , [41] . We tested our data for many semantic similarity thresholds and annotation sets (human, zebrafish, whole UniProt) to take this factor fully into account ( Supplementary Data 1 ). By bootstrapping, we further tested the sensitivity of both the GO and PPI data sets to the influence of a small number of proteins with many annotations. High bootstrap values in almost every case support our conclusions ( Supplementary Data 1 and 2 ). Finally, use of predicted protein interactions can help overcome the lack of PPI information in species outside a few genomic models [47] , [51] . Another approach would be the use of PPI information from well-defined interactomes as gene pleiotropy estimates are based on PPI number, which seems to be an evolutionarily conserved metric in interologous networks [52] . We employed both strategies by counting PPIs either as high-quality experimentally observed annotations assigned to human orthologues or as predicted for zebrafish ( Supplementary Fig. 7 and Supplementary Data 2 ). To avoid incorrect orthologue identification, we used a rather conservative E -value threshold for blastp (≤3.00E−18). All results corroborated that PPI, a proxy for gene pleiotropy, constrain both plastic and evolutionary gene expression responses ( Figs 4 and 6 , Supplementary Figs 3 and 4 and Supplementary Data 2 ). Associating the observed gene expression profiles with upstream regulators links our observations at the molecular level with a phenotypic trait, larval growth, which has been shown earlier to undergo temperature-driven adaptive evolution in this study system [32] , [33] . Myc-target genes are evolutionarily conserved from teleost fishes to mammals and have functional roles for the control of growth during embryonic development via cell proliferation and differentiation [53] . hsf1 is known as the master regulator of the heat-shock response in vertebrates and hsf2 modulates its activity [54] , [55] . Heat-shock regulators are an integral part of the heat-shock response, which has been used to evaluate the acclimation ability and thermal tolerance of species in light of climate change [55] . Many factors can influence protein turnover to regulate protein expression levels inside the cells [56] , [57] but the transcription factor analysis described here provide insights into the larger biological role of the studied proteins. Given our findings, we suggest that the level of pleiotropy of a given gene should have a much more central role when interpreting the biological meaning of gene expression data. Not all proteins seem to have the same capacity to change their expression level as our study shows that proteins with fewer interactions (also more peripheral in the interactome) or involved in fewer biological processes have greater plastic and evolutionary responses to temperature. Accordingly, those low-pleiotropic proteins were driving the observed differences in the global expression profiles. Limitations surrounding gene expression interpretations based on fold-change cut-offs and the corresponding tests have been described [58] , [59] , but a method that takes into account gene pleiotropy could prove valuable for interpretation of gene expression profiling studies in the future. For example, pleiotropic level could be used to weigh the significance of expression-level change, with higher weight being given to changes in genes with higher pleiotropy. Further, we anticipate our findings to serve as a starting point to answer many exciting new questions posed by evolutionary and molecular biologists; for example, are the constraints imposed by gene pleiotropy different at the proteome and transcriptome levels [60] ? This question is important given the discordance between changes in protein and mRNA expression levels [61] , [62] . At the proteome level, we have shown that gene pleiotropy constrains both plastic and evolutionary gene expression responses. At the transcriptome level, previous results have revealed that protein interactions constrain gene expression variation and gene expression divergence between species [31] . The degree of overlap between these findings remains unclear. Pleiotropic constraints may also play a role in various aspects of gene expression control [61] , [63] ; for instance, they may influence translation and transcription rates that in turn have been found to be good predictors of protein expression levels [61] . Furthermore, follow-up studies to clarify associations between expression changes in specific proteins and their effects on fitness-related traits would also be worthwhile. Other intriguing questions include: how are pleiotropic constraints affected by the modularity of biological networks [20] or by tissue specificity [44] ? What is the relative importance of gene pleiotropy for plastic and evolutionary or adaptive responses over longer evolutionary periods? Answering such questions will help further elucidate the role of gene expression regulation in evolution and allow for a better understanding of the molecular basis of adaptation. Sample collection and common garden experiment Full details are available in Thomassen et al . [33] and Haugen and Vøllestad [64] . Animal sampling and experimentation were performed in compliance with the recommendations of the Norwegian Animal Research Authority (permission ID 2008/7368.5). Briefly, samples were obtained from grayling spawning sites from four sub-populations in Lesjaskogsvatnet ( Fig. 1 ). The mean summer, June–July, temperatures in the four streams investigated here differ strongly, with the two small and warm streams, Steinbekken and Sandbekken, being approximately 1–1.5 °C warmer than the large and cold streams, Hyrjon and Valåe (Sandbekken 8.44±0.52 °C ( n =4 years); Steinbekken 8.81±0.60 °C ( n =4); Hyrjon 7.40±0.94 °C ( n =8); Valåe 7.28±0.69 °C ( n =7)). This results in a large temperature-sum difference among streams during egg and larvae development. Developing embryos in the cold streams experience more time at or below 6 °C compared with the warm streams where embryos are subjected to temperatures of 9 °C or higher for longer periods ( Supplementary Table 1 ). In June 2007, adult grayling were captured at the four spawning sites using fyke nets and stripped of gametes, which were subsequently transported on ice to the Veterinary Institute of Norway, Oslo (5 h drive). Gametes were stripped on 12 June 2007 for the warm sites and on 23 June 2007 for the cold sites. This time difference exemplifies the difference in the thermal environments of the streams (time taken to reach the minimum water temperature for spawning). Samples were the product of artificially fertilized gametes of multiple individuals per sub-population (Steinbekken 20♀, 16♂; Sandbekken 17♀, 11♂; Hyrjon 4♀, 3♂; Valåe 20♀, 24♂). Fertilized eggs were placed in porous containers suspended in the large treatment tanks as described previously [33] , [64] . Each of the tanks contained two replicate containers from each sub-population. The water temperatures of the cold and warm temperature treatments across the experiment were 5.83±0.43 °C ( n =764) and 10.02±0.28 °C ( n =440), respectively, to represent lower and upper temperatures experienced by developing grayling larvae in nature [33] ( Supplementary Table 1 ). Each day post fertilization, approximately five individuals (eggs or larvae) were randomly sampled from each sub-population in each temperature treatment. Samples were visually inspected and whether an individual had hatched or not was recorded. Samples used for the proteomics experiment were immediately frozen on dry ice and transferred to −80 °C within ~30 min for storage. Grayling embryos selected for protein extraction were of similar developmental stage as estimated based on the number of degree-days (temperature in °C × number of days elapsed since fertilization) in relation to the average number of degree-days to 50% hatching in the sub-population—temperature treatment ( Supplementary Table 3 ). The effect of thermal origin on the number of degree-days to 50% hatching was tested by performing a binomial logistic regression using a generalized linear model. The generalized linear model was performed with a logit link function and with the count of the hatched and not-hatched individuals per sampling day as the dependent variable, and the number of degree-days and thermal origin as independent variables. Degree-day values for a 50% probability of hatching for each experimental group and s.e. were estimated using the dose.p function from the MASS library in R [65] . Measuring protein expression levels Details about the protein extraction, peptide-level iTRAQ labelling, fractionation by isotope coded affinity tag procedure, liquid chromatography–tandem mass spectrometry and protein quantification parameters can be found in the Supplementary Methods . The mass spectrometry files (*.RAW), the processed peaklists (*.mgf), the search databases (*.fasta) and the results of the ProteinPilot searches (*.xml) for both the validation and the actual experiment have been deposited in the ProteomeXchange consortium ( http://proteomecentral.proteomexchange.org ) via the PRIDE partner repository [66] with the data set identifier PXD000368. Three embryos per sub-population per common garden temperature treatment, 24 samples (that is, 3 embryos × 4 sub-populations × 2 temperature treatments), were labelled by iTRAQ, fractionated by strong cation exchange chromatography and combined accordingly to minimize batch effects ( Supplementary Table 5 ). Protein identification and quantification were done using the ProteinPilot v.4 programme (Applied Biosystems). As a search database, we used all Atlantic salmon ( Salmo salar ) submitted in the UniProt database ( www.uniprot.org ) as of March 2012 (13,035 amino acid sequences). Maximum false discovery rate correction for protein identification was performed using a decoy database as implemented in ProteinPilot and was set to 5%, whereas minimum confidence for peptide identification was 95%. A collection of 248 sequences of common-contaminant proteins, provided by Applied Biosystems, was also included in the search database. Contaminant and decoy hits were filtered and samples were divided into four groups of six samples each, namely the grayling embryos from each of the cold/warm thermal origin with each of the 6 °C/10 °C temperature treatments. Proteins were also filtered for missing values so that each group had at least three valid ratios. Ratios were then log 2 -transformed and then loess-normalized across biological replicates using the median values as a reference set. For these transformations, we used DanteR, an R package for the analysis of proteomic data (updated edition of DAnTE [67] ). The accuracy of the quantification method was evaluated using a six-protein mix provided with the iTRAQ kit ( Supplementary Methods , Supplementary Fig. 8 and Supplementary Data 3 ). Statistical analyses R scripts for all statistical analyses are available in Supplementary Data 4 . All GLMM analyses verified the assumptions required for linear modelling between dependent variables and continuous predictors, namely normal distribution of the residuals, and the absence of strong heteroscedasticity ( Supplementary Figs 9 and 10 ). To test the effect of thermal origin (cold versus warm sub-populations), temperature treatment (6 °C versus 10 °C) and their interaction on the protein expression profiles, we used the coordinates of normalized expression ratios ( Supplementary Data 5 ) along the first component (PC1) of a PCA. We used PCA because it inherently focuses on summarizing the differences in expression between thermal origins and temperature treatments, without the need to standardize for the direction of change in expression for each protein in every sample. Next, a GLMM analysis was performed with the PC1 coordinates as a dependent variable. Thermal origin, temperature treatment and their interaction were used as independent, categorical, fixed factors and sub-population as a random factor ( Supplementary Methods ). Hierarchical clustering was performed directly on the log 2 -transformed and loess-normalized data using Euclidean distances. Gene expression data were visualized as heatmaps. Q ST − F ST comparisons were made to assess the role of divergent selection in protein expression divergence betweeen sub-populations. F ST was calculated using Weir and Cockerham’s θ (theta) and Q ST was calculated using the formula σ 2 GB / ( σ 2 GB +2 σ 2 GW ), where σ 2 GB is the among sub-population and σ 2 GW is the average within sub-population component of protein expression variance in each temperature treatment [68] . Variance components for every protein were estimated using a restricted maximum likelihood approach, with sub-population as a random factor. By repeating this procedure for all of the proteins in both temperature treatments ( N =408+408, because of the two temperature treatments), we obtained the Q ST distributions [68] . F ST was estimated using data for 19 microsatellites genotyped at 38–44 individuals per sub-population (data from Junge et al . [35] where the sub-populations are labelled STE07: Steinbekken, SAN07: Sandbekken, SHYR08: Hyrjon and VAL07: Valåe). Weir and Cockerham’s F ST can produce slightly negative estimates, thus any negative values of F ST were adjusted to zero; hence, F ST had the same range as Q ST . The F ST sampling distribution was estimated from 1,000 resamples with the hierfstat R package [69] , using similar sample size to that used in Q ST estimations ( n =3 per population). The upper 95% confidence interval of the F ST sampling distribution was set as the threshold for the neutral divergence expectation to quantify the outlier Q ST estimates. χ 2 -test was used to test whether the number of outliers significantly exceeded what may be expected by chance alone. The common garden rearing of fish ensures environmental effects do not inflate the among-sub-population variance, which is a major source of bias in Q ST estimation [17] . Other factors, for example, maternal, epistatic and dominance effects, may bias Q ST estimation, but usually downwards, by upwardly biasing additive genetic variance [68] , thereby making the test of divergent selection applied here a conservative one. Similarly, mutations might bias Q ST estimates downward through increased dominance variance [17] ; however, due to the low divergence times, mutations are not expected to play a large role in the evolution of this system. To test the effect of gene pleiotropy on protein expression responses, we first studied the mean standardized expression of grouped proteins. A GLMM was applied using all 408 quantified proteins with loess-normalized and log 2 -transformed values ( Supplementary Data 5 ). Standardized protein expression level was the dependent variable, and the independent variables were as follows: thermal origin (categorical), temperature treatment (categorical), gene pleiotropy (continuous) and their interactions (fixed effects). Sub-population and individual were used as random factors. Sub-population was nested within thermal origin and individuals were nested within sub-population. Raw gene pleiotropy value distributions were initially strongly skewed and therefore log 2 -transformed. To fulfil the assumptions of GLMM of the dependent variable (reduce kurtosis) and reduce the complexity of the GLMM, proteins were grouped based on level of pleiotropy. This was done by ordering the proteins according to their pleiotropy level (the ordering varied depending on what measure of gene pleiotropy, PPI or GO-BP, was used each time), with random order within each level of pleiotropy and subsequently dividing the ordered proteins into groups of ten. GLMM analysis was repeated for group sizes ranging from 2 to 30 and group size=10 represented a good compromise between minimizing the kurtosis while retaining the groups as small as possible to have more data points in the analyses ( Supplementary Fig. 11 ). Bin size had little effect on the observed P -values and the results were also highly significant if no binning was used ( Supplementary Data 1 and 2 ). For each group of proteins, we calculated the average value for log 2 (pleiotropy+1) and the average standardized protein expression level for each individual and used these data in the GLMM. In this way we avoid side effects of unequal group sizes, which would arise if we had simply grouped by the pleiotropy level. For comparison, we also did the analysis without grouping the proteins. As the analysis of the effect of gene pleiotropy focused on the extent of expression change, and not the direction (increase or decrease in expression), we standardized protein expression values by removing differences in the direction of the expression change between proteins as follows: we used the experimental group with the largest differential response in the PCA as a reference (Valåe at 6 °C, Fig. 3 ) and whenever the median expression level of a protein in this reference population (median over three replicate individuals) was below the overall median expression level (median over 24 individuals), we flipped the individual expression levels around the overall median expression level for that protein. By using the median expression level within one reference sub-population and flipping the sign of expression level for all individuals in the entire data set when needed, we conserve the independence of the values between the 24 individuals needed for statistical inference, but eliminate between-protein differences in the direction of the expression change. In a second approach, we tested the effect of gene pleiotropy on protein expression responses using the mean standardized expression of the 30% most variable proteins per group of ten proteins ( Supplementary Methods ). With this approach we excluded the contribution of proteins in our data set that are less likely to be linked to temperature responses, that is, those that had low levels of expression variation, and therefore we increased the power to detect differences between thermal origins and temperature treatments. In a third approach, we tested the effect of gene pleiotropy on protein expression responses by performing multidimensional scaling analysis ( Supplementary Methods ). We used this approach as an alternative to reduce the influence of non-responsive proteins within each level of gene pleiotropy and increase the power of our analysis. This is because the scores from the multidimensional scaling analysis are mainly determined by the subset of proteins that show strong differential protein expression response. Therefore, this approach focuses more on those proteins. Estimating gene pleiotropy Gene pleiotropy was estimated either as the amount of known PPI or GO terms [27] . GO terms were retrieved separately for GO-BP, GO-CC and GO-MF. For each of these measures we performed an independent analysis. PPI counts and GO annotations were retrieved from human ( Homo sapiens ) orthologues of the detected salmonid proteins. Orthologues were identified by sequence similarity with blastp using the human reference proteome in UniProt ( www.uniprot.org , version 10 June 2013) as the search database and a minimum E -value of 3.00E−18 ( Supplementary Data 6 and 7 ). The more comprehensive annotation for H. sapiens genes often makes them preferred even over zebrafish for the transfer of annotations to fish species; however, we also conducted an analysis based on zebrafish data, which is currently among the best annotated fish species. GO annotations for the human genes were downloaded from the GO website ( www.geneontology.org , version 6 June 2013). PPI were retrieved from the Ingenuity Pathway Analysis (IPA 2013) platform and included only experimentally observed direct interactions in the BIND, BIOGRID, Cognia, DIP, INTACT, MINT and MIPS databases, as well as Ingenuity expert findings as of 17 June 2013. Annotation bias, particularly in human GO annotations, can occur because the discovery of new processes or functions is less frequent than the proliferation of semantically similar GO terms [39] . For this reason, we also summarized semantically similar GO terms and re-analysed the data to determine whether redundancy has a marked effect on our findings. Redundancy was treated with REVIGO using SimRel as a semantic similarity measure [42] . We examined three different levels of allowed similarity, namely large (allowed similarity=0.9), medium (0.7), which is the default option in REVIGO, and small (0.5). We also ran all our analyses with three different GO databases (whole UniProt, H. sapiens and D. rerio ) to estimate the information content of each term during the calculation of the semantic distances. This was done separately for each protein and for GO-BP, GO-MF and GO-CC ( Supplementary Data 6 ). Bootstrap test To test the robustness of our GLMM analyses, we repeated all of the analyses on each of 2,000 bootstrap re-samples (except for standardized protein expression levels without grouping that was very computer-intensive for which we used 100 bootstrap re-samples). Each re-sample was generated by randomly sampling the 408 proteins from the original data set with replacement. The bootstrap values were then calculated as the proportions of re-sampled data sets for which the analyses yielded a significant P -value<0.05 ( Supplementary Data 1 and 2 ). PPI proxies for zebrafish To corroborate the results obtained with experimentally observed PPI in human orthologues, we looked for predictors of PPI in zebrafish. We used Funcoup 2.0, which applies an optimized Bayesian framework to reconstruct global networks of protein functional coupling (FC) by integrating proteomic and genomic data from multiple species [47] , [51] . Data files for human and zebrafish were retrieved from the Funcoup server and each final Bayesian score (FBS) was converted to a probability of FC (pfc) using pfc=1/(1+exp(−FBS— ln ( P (FC)))) where P (FC)=0.001 (ref. 47 ). In all analyses using the Funcoup database, we considered only interactions with pfc>0.9 for the category of interest to ensure only high-quality interactions were included ( Supplementary Methods and Supplementary Data 7 ). The effect of genes with contrasting pleiotropy levels To assess how proteins with lower or higher pleiotropy drive the differences in expression profiles between experimental groups, we conducted a post-hoc analysis as follows: we used the median value of PPI and GO-BP to separate the proteins into two groups with low or high PPI and GO-BP counts (PPI: median=51, low PPI group: 120 genes, high PPI group: 119 genes; GO-BP: median=10.5, low PPI group: 122 genes, high PPI group: 122 genes). PCA and hierarchical clustering were re-performed on those sub-sets of proteins with low or high pleiotropy, and the PC1 coordinates were then used in a GLMM with thermal origin, temperature treatment and their interaction as independent fixed factors, and sub-populations as random factors nested within thermal origin ( Fig. 5 , Supplementary Fig. 5 and Supplementary Table 6 ). For this analysis we used the 244 proteins with no missing values. Upstream regulator analysis To identify upstream regulators that explain the observed gene expression changes, we used the IPA platform. IPA examines every known upstream regulator for each gene in our data set and compares the observed direction of change in protein expression with that expected based on literature findings stored in the IPA knowledgebase. Significant activation or inhibition of an upstream regulator is predicted based on evidence from multiple target genes in the data set for which the direction of the observed expression change is consistent with that expected from the literature. To calculate the direction of expression change for each protein, we used the median values across all six biological replicates per thermal origin-temperature treatment combination. Z -score value specifies whether an upstream regulator has significantly more activated predictions than inhibited predictions ( Z >2) or vice versa ( Z <2). The bias metric estimates whether there are more up- than downregulated genes or vice versa for an upstream regulator in the data set (there should be enough evidence from both directions for reliable predictions). Overlap P -value is calculated using Fisher’s exact test and determines whether there is a statistically significant higher presence of genes controlled by an upstream regulator in the data set compared with a reference list of genes. In our case, we used the gene list of the Agilent zebrafish V2 microarray, which represents the genome of the teleost species D. rerio [70] . To add specificity to our analyses, we considered only direct and experimentally observed molecular interactions. We only examined the most reliable predictions, as recommended by IPA Systems ( P <0.001, | Z |>2, and bias|<0.25). Details about the employed algorithms are described elsewhere [48] . How to cite this article: Papakostas, S. et al . Gene pleiotropy constrains gene expression changes in fish adapted to different thermal conditions. Nat. Commun. 5:4071 doi: 10.1038/ncomms5071 (2014).